Electronic metal-support interactions in vacuum vs. electrolyte First, we like to clarify that the potential of zero charge (pzc) that we have referred to in our original communication is distinct from the potential where the nanoparticles have zero charge that is the subject of Binninger’s consideration. The diagram of Fig. 1 shows a simplified sketch of the charging behaviour of the nanoparticles and support. Following Binninger’s assumptions, we only consider here electrostatic interactions and assume that the charging is purely capacitive and linear in potential following the commonly used model from Bockris et al. [6] . This might not be justified in general as we will point out below, but it is useful to understand the implications of Binninger’s assumptions. Fig. 1: Idealised sketch of the potential of zero charge of a heterogeneous electrode. Shown are linearised charging curves per total surface area for support and nano-particle as a function of potential; the overall pzc is defined by equal but opposite charges on support (line AC) and nano-particle (line BC). Full size image The nano-particle and support, in general, have different work functions. Hence, they will exchange charge until their Fermi levels are equilibrated when brought into contact with the forming dipoles resulting in a coverage-dependent change of overall work function [7] and corresponding overall pzc. Under overall charge neutrality and assuming that charging across the direct catalyst-support interface is fully separable from charging across the electrolyte-facing interfaces, the magnitude of charge transferred from the support surface (line AC in Fig. 1 ) to the nanoparticle surface (line BC in Fig. 1 ) has to be equal at the pzc of the overall electrode. This clearly is a function of the support material and distinct from the potential where the catalyst nanoparticles have zero charge. 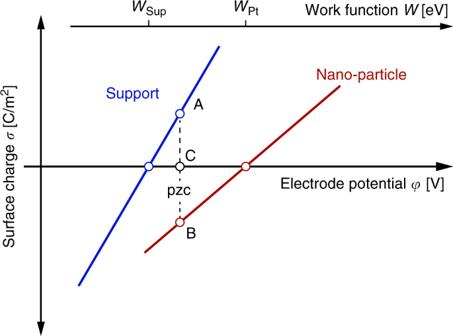Fig. 1: Idealised sketch of the potential of zero charge of a heterogeneous electrode. Shown are linearised charging curves per total surface area for support and nano-particle as a function of potential; the overall pzc is defined by equal but opposite charges on support (line AC) and nano-particle (line BC). Figure 1 suggests that a lower work function of the support should shift the pzc towards more negative potentials, but the implied linear relationship could be an oversimplification. It is, therefore, valid to ask if the overall work function (and consequently the pzc) would also be framed by the work functions of the support and catalyst nanoparticle more generally. The overall work function of similar heterosystems has been shown theoretically [7] and experimentally [8] to fall in-between the work functions of the support and nanoparticle, giving us reason to believe that this relationship holds qualitatively more generally. As we have pointed out in our original communication and clarified above, this shift of pzc implies a more positive charge for the electrode with the lower work function support if the electrodes are held at the same potential. However, the question remains, how the additional charge is distributed across the catalyst and support? An important consequence of assuming full screening through the electrolyte is that the charge on the Pt nanoparticles as a function of voltage would be independent of the support material, not only at the potential where the nanoparticles carry zero charge as pointed out by Binninger, because the charge–voltage curve is the same for the nanoparticles in contact with the support and without. In contrast, our experimental results indicate that a larger fraction accumulates at the nanoparticles, but a general theoretical understanding of the charge distribution away from the pzc eludes us so far. Chemical and electrostatic interactions with the electrolyte and/or the electronic structure of catalyst and support could all be important factors. We stress that the reasoning above reflects a highly idealised situation. As we have communicated recently elsewhere [9] , the charging behaviour of the Pt nanoparticles supported on BC as a function of voltage in acidic electrolyte is markedly different from the Pt nanoparticles supported on C. The electronic structure of Pt nanoparticles supported on BC and C was probed using XANES over a range of potentials. These experiments showed that at moderate potentials (below approximately 0.9 V vs. RHE), the Pt/BC catalyst has a higher d-band vacancy density than the Pt/C catalyst, while at higher potentials above 0.9 V vs. RHE the Pt/C catalyst showed more vacancies in the Pt d-band manifold, providing direct experimental evidence for a change of sign of the relative d-band filling between the two catalysts depending on potential. Unfortunately, the situation is complicated by chemical interactions between catalyst and electrolyte at high potentials, and the relative trends in d-band vacancy should not be directly correlated with the state of charge of the nanoparticles at high potentials, as partial oxidation of the nanoparticles will contribute as well. The complex charging behaviour of Pt in aqueous electrolyte has recently been investigated in great detail by Eikerling and co-workers [10] using a quantitative model that goes beyond that discussed by Binninger. They could show that the charging behaviour of metallic Pt cannot be assumed to be monotonic in aqueous electrolyte and that there is no unique potential of zero charge of metallic Pt due to the complexity of the interactions between Pt and aqueous electrolytes. Finally, we like to comment on Binninger’s assertion that “the majority of transferred charge is accumulated at the direct support-Pt interface and, therefore, unaffected by the external environment”. As we recently communicated elsewhere [9] , we used potentiostatic CO displacement measurements [11] to estimate the surface charge of the Pt nanoparticles in electrochemical environments. Unfortunately, these measurements cannot be used to directly obtain the pzc, partially due to the common occurrence of charge-transfer chemisorption to form adsorbed hydrogen [12] . However, these measurements have shown displacement charges of about 60 μC/cm Pt 2 for Pt/BC and 20 μC/cm Pt 2 for Pt/C, respectively, in the double layer region (potentials of about 0.3 to 0.6 V vs. RHE) where chemisorbed hydrogen is unlikely to occur. Estimates for the pzc of extended Pt electrodes vary, but usually range from close to 0 V vs. SHE [12] to values closer to 0.25 V vs. SHE [13] . Regardless, Pt electrodes in the electrolyte used (0.1 M HClO 4 ) are typically reported to have a capacitance of around 15 μF/cm Pt 2 [11] , [12] , [13] , which would suggest surface charges no larger than 10 μC/cm Pt 2 in the double layer region for unsupported Pt electrodes. Geometric effects [14] might contribute to the larger capacitance of the supported catalysts relative to the expected capacitance of unsupported Pt, but are less relevant for the comparison of Pt/BC and Pt/C given their similar geometries. We, therefore, take the larger displacement charge of Pt/BC relative to Pt/C as an indirect indication of a shift of the pzc towards lower values for Pt/BC compared to Pt/C and further experimental evidence that electronic metal support interactions in electrochemical environments are not largely confined to the direct catalyst-support interface as conjectured by Binninger, but have bearings on the electrochemical properties of the catalyst-electrolyte interface. The dependence of CO stretching modes on local electric fields [15] might provide convenient spectroscopic probes (e.g., through Infrared Reflection−Absorption Spectroscopy or Sum-Frequency Vibrational Spectroscopy [16] ) to further study these surface charge effects.